p53 regulatesPeriod2expression and the circadian clock The mechanistic interconnectivity between circadian regulation and the genotoxic stress response remains poorly understood. Here we show that the expression of Period 2 (Per2) , a circadian regulator, is directly regulated by p53 binding to a response element in the Per2 promoter. This p53 response element is evolutionarily conserved and overlaps with the E-Box element critical for BMAL1/CLOCK binding and its transcriptional activation of Per2 expression. Our studies reveal that p53 blocks BMAL1/CLOCK binding to the Per2 promoter, leading to repression of Per2 expression. In the suprachiasmatic nucleus (SCN), p53 expression and its binding to the Per2 promoter are under circadian control. Per2 expression in the SCN is altered by p53 deficiency or stabilization of p53 by Nutlin-3. Behaviourally, p53 −/− mice have a shorter period length that lacks stability, and they exhibit impaired photo-entrainment to a light pulse under a free-running state. Our studies demonstrate that p53 modulates mouse circadian behaviour. It is recognized that circadian function and the genotoxic stress response are interconnected. This is thought to be an evolutionary adaption of the organism to sunlight irradiation on earth. The transcription factor p53 is known as the ‘guardian of the genome’ [1] , [2] . The majority of all human tumours have mutations in the TP53 gene, which encodes the p53 protein [3] . The roles of stress-induced p53 in cellular responses are well studied. For example, cell cycle arrest and the DNA damage response are among the biological processes that are regulated by stress-induced p53 (ref. 4 ). Circadian rhythms are the daily oscillations of biological processes driven by endogenous molecular clocks [5] . The known core clock genes include Clock, Npas2, Bmal1, Per1, Per2, Cry1, Cry2, CK1ε, CK1δ, Rev-Erbα and RORα. Typically, the BMAL1/CLOCK heterodimer binds to the E-box in the promoter region of their target genes, leading to activation of the expression of these genes, including Per1, Per2, Cry1 and Cry2 . The protein products of these core clock genes regulate each other’s expression in the feedback loops. Recently, we showed that the promyelocytic leukaemia (PML) protein regulates the circadian clock by interacting with PER2 and enhancing BMAL1/CLOCK-mediated transcription [6] . PML is essential for the formation of PML nuclear bodies (NBs) [7] . It is thought that PML-NBs recruit specific proteins and regulate their activity by modulating their post-translational modification. To date, a growing list of PML-interacting proteins has been reported [8] . Among them are both positive and negative regulators involved in the circadian clock mechanism including PER2, BMAL1, SIRT1, CBP, WDR5 and SIN3A [6] , [9] , [10] , [11] , [12] . These findings led us to screen other PML-associated proteins for a possible role in modulating BMAL1/CLOCK-mediated Per2 transcription. Among the PML-associated proteins examined was p53, which is known to localize with the PML-NB. Studies have shown that acetylation and deacetylation of p53 by CBP and SIRT1, respectively, are PML-NB-dependent [13] , [14] , [15] . Here, we show that p53 modulates the circadian behaviour of mice by modulating Per2 expression, acting as a direct competitor of BMAL1/CLOCK binding to the Per2 promoter. This mechanistic interaction may represent a key regulatory link between the p53-mediated cellular stress response and the circadian clock-regulated cellular pathways. p53 represses BMAL1/CLOCK-mediated transcription of Per2 A number of PML-associated proteins were screened for their potential ability to modulate BMAL1/CLOCK-mediated Per2 promoter transcription. Expression constructs for p53, WRN, RB and RARα were individually examined using a Per2-Luc reporter assay for their ability to upregulate or downregulate BMAL1/CLOCK-mediated transcription. Among these expression constructs, we observed that the one encoding p53 strongly repressed BMAL1/CLOCK-mediated transcription of the Per2 promoter ( Fig. 1a ). Therefore, we asked whether this apparent repression of Per2 transcription by p53 was mediated through BMAL1/CLOCK. High levels of p53 can induce apoptosis of tumour cell lines and this could result in an apparent nonspecific transcriptional repression [16] . To rule out this possibility, we compared wild-type mouse embryonic fibroblasts (MEFs) with HeLa cells using a Luc-reporter assay driven by either the Bmal1 or Per2 promoter. In both wild-type MEF and HeLa cells, the expression of p53 did not repress RORγ-mediated transcription of the Bmal1 promoter but repressed Per2 promoter transcription mediated by BMAL1/CLOCK ( Fig. 1b and Supplementary Fig. S1 ). 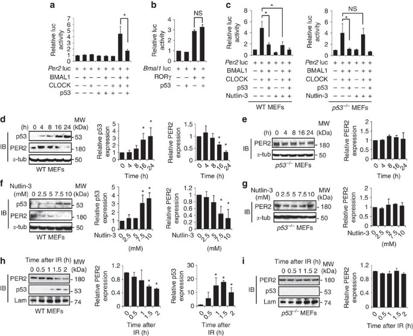Figure 1: p53 modulatesPer2expression. (a)Per2or (b)Bmal1promoter luciferase assay in wild-type (WT) MEF cells transfected with the indicated expression vectors and harvested 24 h after transfection. (c)Per2promoter luciferase assays in the absence or presence of Nutlin-3 (10 μM) using WT orp53−/−MEF cells. Western blotting using the indicated antibodies; (d) WT or (e)p53−/−MEF cells were treated with 10 μM Nutlin-3 and harvested at the indicated time points; (f) WT orp53−/−(g) MEF cells were treated with the indicated concentration of Nutlin-3 for 16 h. (h) WT or (i)p53−/−MEF cells were treated with γ-irradiation (10 Gy) and harvested at the indicated time points (full-length immunoblots images for d and h are shown inSupplementary Fig. S8). Error bars; mean±s.e.m. (n>3).t-Test: *P<0.05. NS, not significant. Figure 1: p53 modulates Per2 expression. ( a ) Per2 or ( b ) Bmal1 promoter luciferase assay in wild-type (WT) MEF cells transfected with the indicated expression vectors and harvested 24 h after transfection. ( c ) Per2 promoter luciferase assays in the absence or presence of Nutlin-3 (10 μM) using WT or p53 −/− MEF cells. Western blotting using the indicated antibodies; ( d ) WT or ( e ) p53 −/− MEF cells were treated with 10 μM Nutlin-3 and harvested at the indicated time points; ( f ) WT or p53 −/− ( g ) MEF cells were treated with the indicated concentration of Nutlin-3 for 16 h. ( h ) WT or ( i ) p53 −/− MEF cells were treated with γ-irradiation (10 Gy) and harvested at the indicated time points (full-length immunoblots images for d and h are shown in Supplementary Fig. S8 ). Error bars; mean±s.e.m. ( n >3). t -Test: * P <0.05. NS, not significant. Full size image The endogenous p53 level is stabilized and enhanced by Nutlin-3, a small-molecule inhibitor of MDM2 (ref. 17 ). MDM2 is the major negative regulator of p53 and facilitates p53 degradation [18] . BMAL1/CLOCK-mediated transcription of the Per2 promoter was repressed in wild type, but not in p53 −/− MEF cells, when treated with Nutlin-3 ( Fig. 1c ). Transfection of a p53 expression construct into p53 −/− MEF cells restored the repression of BMAL1/CLOCK-mediated transcription of the Per2 promoter in the presence of Nutlin-3. Western blot analysis with anti-p53 and anti-PER2 antibodies showed a time-dependent increase in the levels of endogenous p53, accompanied by a reciprocal decrease in endogenous PER2 in wild-type MEF cells following Nutlin-3 treatment ( Fig. 1d ). No decrease in PER2 levels by Nutlin-3 treatment was observed in p53 −/− MEF cells ( Fig. 1e ). This inverse relationship between p53 and PER2 levels was further examined in a Nutlin-3 titration experiment. After a 16-h treatment, endogenous p53 levels correlated with increases in Nutlin-3 concentration, and were inversely correlated with PER2 levels in wild-type MEF cells ( Fig. 1f ). No change in PER2 levels was observed when p53 −/− MEF cells were treated with Nutlin-3 at a similar concentration ( Fig. 1g ). Genotoxic stress such as γ-irradiation is known to rapidly stabilize p53 protein in some cells, including MEF and human osteosarcoma U2OS cells [19] . Western blot analysis of human U2OS cells and wild-type MEF treated with γ-irradiation displayed a rapid rise in p53 and a reciprocal decline in PER2 levels ( Fig. 1h , Supplementary Fig. S2 ). This decline in PER2 level was not observed in p53 −/− MEF cells that were similarly treated with γ-irradiation ( Fig. 1i ). Together, these studies show that the cellular level of PER2 is inversely correlated with that of p53. The Per2 promoter contains a conserved p53 response element The inverse correlation between p53 and PER2 suggests that p53 is repressing BMAL1/CLOCK-mediated transcription of the Per2 promoter. To map the putative response element for p53 , BMAL1/CLOCK-mediated transcription reporter assays were carried out using serial deletion constructs of the mouse Per2 promoter between −2,811 and −105 bp from the transcription start site ( Fig. 2a ). The repression by p53 of BMAL1/CLOCK-mediated transcription of the Per2 promoter was intact in all of these deletion constructs suggesting that the putative p53 response element is within the −105 bp region of the Per2 promoter. Using the NBLAST programme, comparison of this 105 bp mouse sequence with Per2 promoter sequences of human, dog and rat from Genebank revealed a highly conserved 48 bp sequence ( Fig. 2b ). Sequence analysis with the TFBIND programme revealed a putative p53 response element. The p53 response element is a motif of two tandem decamers separated by 0–13 nucleotides. The consensus sequences can be depicted as 5′-RRXCXXGXYX-N(0–13)-XRXCXXGXYY-3′, where R=A/G, Y=C/T and X=A/G/C/T [20] . This putative p53 response element is upstream to the transcription start site of the Per2 promoter, and its proximal decamer overlaps with the critical E-box sequence for BMAL1/CLOCK binding. Mutation of nucleotides adjacent to the E-box severely dampened BMAL1/CLOCK-mediated transcription of the Per2 promoter. These observations are consistent with previous findings that BMAL1/CLOCK-mediated transcription of the Per2 promoter requires a segment ~20 bases from the transcription start site [21] . Interestingly, mutation of nucleotides in the distal decamer of the putative p53 response element did not significantly affect BMAL1/CLOCK-mediated transcription, whereas the strong repression by p53 was relieved ( Fig. 2b,c ). 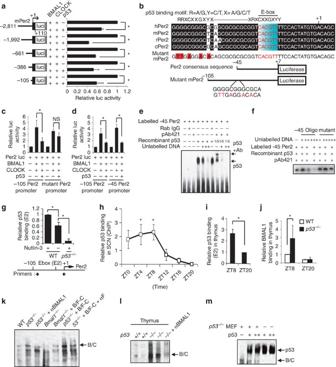Figure 2: p53 binds to aPer2promoter consensus region. (a)Per2promoter deletion luciferase assay. (b) Comparison ofPer2promoter among species (upper). Images of −45 bp WT and mutantPer2promoter luciferase construct (lower). Luciferase assays were performed using: (c) −105 bp WT and mutantPer2or (d) −105 bp and −45 bpPer2promoter luciferase. (e) p53 binding to thePer2promoter consensus region examined by EMSA. (f) Competition assay for p53 binding by EMSA. (g) Relative p53 binding to thePer2promoter (E2) was examined by ChIP–qPCR assay. (h) ChIP–qPCR assay for p53 in mouse SCN. ANOVA:P<0.05,post hoc t-test: *P<0.05. (i) ChIP–qPCR assay (E2) for p53 in mouse thymus. (j) ChIP–qPCR assay (E2) for BMAL1 in wild-type (clear) or p53−/−(shaded) mouse thymus obtained at ZT8 and ZT20. (k) BMAL1/FLAG-CLOCK (B/F-C) binding to thePer2promoter consensus region examined by EMSA. Nuclear extracts from the indicated genotype of fibroblast cells were used. (l) EMSA of BMAL1/CLOCK (B/C) binding using nuclear extract obtained from the thymus. (m) Competitive binding assay to thePer2promoter by EMSA using recombinant p53 and BMAL1/CLOCK from nuclear extract ofp53−/−MEF cells. Error bars: mean±s.e.m. (n>3).t-Test: *P<0.05. NS, not significant. Figure 2: p53 binds to a Per2 promoter consensus region. ( a ) Per2 promoter deletion luciferase assay. ( b ) Comparison of Per2 promoter among species (upper). Images of −45 bp WT and mutant Per2 promoter luciferase construct (lower). Luciferase assays were performed using: ( c ) −105 bp WT and mutant Per2 or ( d ) −105 bp and −45 bp Per2 promoter luciferase. ( e ) p53 binding to the Per2 promoter consensus region examined by EMSA. ( f ) Competition assay for p53 binding by EMSA. ( g ) Relative p53 binding to the Per2 promoter (E2) was examined by ChIP–qPCR assay. ( h ) ChIP–qPCR assay for p53 in mouse SCN. ANOVA: P <0.05, post hoc t -test: * P <0.05. ( i ) ChIP–qPCR assay (E2) for p53 in mouse thymus. ( j ) ChIP–qPCR assay (E2) for BMAL1 in wild-type (clear) or p53 −/− (shaded) mouse thymus obtained at ZT8 and ZT20. ( k ) BMAL1/FLAG-CLOCK (B/F-C) binding to the Per2 promoter consensus region examined by EMSA. Nuclear extracts from the indicated genotype of fibroblast cells were used. ( l ) EMSA of BMAL1/CLOCK (B/C) binding using nuclear extract obtained from the thymus. ( m ) Competitive binding assay to the Per2 promoter by EMSA using recombinant p53 and BMAL1/CLOCK from nuclear extract of p53 −/− MEF cells. Error bars: mean±s.e.m. ( n >3). t -Test: * P <0.05. NS, not significant. Full size image To further characterize the region upstream of the Per2 promoter initiation site, sense and antisense oligonucleotides corresponding to the mouse Per2 promoter sequence from +7 to −45 bp were synthesized, annealed and cloned into a luciferase reporter vector to generate −45 bp Per2 -Luc ( Fig. 2b ). Transcriptional activation by BMAL1/CLOCK and repression by p53 of expression from the −45 bp Per2 -Luc and −105 bp Per2 -Luc reporter constructs were comparable, indicating that the −45 bp Per2 DNA promoter sequence contained both the p53 response element and the E-box of BMAL1/CLOCK ( Fig. 2d ). Using an electrophoretic mobility shift assay (EMSA), we observed that recombinant p53 protein binds to −45 bp Per2 DNA ( Fig. 2e ). The binding of p53 to biotin-labelled −45 bp Per2 DNA was competitively reduced by unlabelled −45 bp Per2 DNA. Some antibodies to p53 are known to induce a super-shift of the p53/DNA complex. We tested two commercial p53 antibodies and they both generated the expected super-shifts ( Fig. 2e , Supplementary Fig. S3 ). Further, the super-shift was competitively reduced by unlabelled −45 bp Per2 DNA. However, when the unlabelled −45 bp Per2 DNA contained a mutated sequence in the distal decamer, the super-shift binding was not reduced ( Fig. 2f ). The Per2 genomic locus has five described E-box elements (E1–E5), and the one most critical for BMAL1/CLOCK binding is E2 located in the promoter region [22] . Chromatin immunoprecipitation (ChIP) assays with anti-p53 antibodies were performed using genomic DNA that had been fragmented to 0.5 Kb on average. ChIP–quantitative (q) PCR analysis revealed that p53 pull-down of E2 was significantly enhanced in wild-type when cells were treated with Nutlin-3 ( Fig. 2g ). In contrast, p53 pull-down of E5, ~3 Kb away from E2, was not significant ( Supplementary Fig. S4 ). Next, we determined whether BMAL1/CLOCK binding to the E2 region of the Per2 promoter was disrupted by p53. Transfection of p53 −/− MEF with expression constructs for FLAG-tagged Clock , Bmal1 in the presence or absence of a p53 expression construct was carried out. ChIP–qPCR analysis showed that in the absence of p53, pull-down of FLAG-CLOCK by the anti-FLAG antibody was significantly higher ( Supplementary Fig. S5 ). We then investigated whether p53 binding to the E2 region of the Per2 promoter also occurs in the SCN in vivo . SCNs from wild-type mouse brains were dissected at six zeitgeber time (ZT) points over 24 h for ChIP analysis. ChIP–qPCR with anti-p53 antibodies showed a peak level of endogenous p53 binding to the Per2 promoter in the SCN between ZT4–ZT8 and a nadir at ZT16–ZT20 ( Fig. 2h ). These studies demonstrate that p53 is expressed in the SCN and its interaction with the Per2 promoter is under temporal control in vivo . Next, the level of p53 or BMAL1/CLOCK binding to the E2 region of the Per2 promoter was examined using wild-type and p53 −/− mouse thymus obtained at ZT8 and ZT20. Thymus was chosen as it expresses detectable levels of p53 under normal physiological conditions. ChIP–qPCR analysis revealed that p53 binding to the E2 region was about 2.5 times higher at ZT8 than at ZT20 ( Fig. 2i ). BMAL1 binding to the E2 region in p53 −/− MEF was significantly elevated compared with wild-type MEF ( Fig. 2j ). To investigate whether p53 directly competes with BMAL1/CLOCK for binding to the −45 bp Per2 DNA, nuclear extracts from WT, p53 −/− MEF and Bmal1 −/− fibroblasts were prepared for EMSA. Unlike nuclear extracts from WT and p53 −/− MEF, those from Bmal1 −/− fibroblasts did not display a prominent protein/DNA complex on EMSA with −45 bp Per2 DNA indicating that this complex is BMAL1 dependent ( Fig. 2k ). Further, transfection of expression plasmids for Bmal1 and Flag-Clock into Bmal1 −/− fibroblasts restored the BMAL1/CLOCK:−45 bp Per2 protein/DNA complex in nuclear extracts. Treatment with either anti-BMAL1 or anti-FLAG antibodies significantly reduced this protein/DNA complex. Consistent with results from ChIP–qPCR analysis, nuclear extracts from p53 −/− MEF and thymus showed an increased level of the BMAL1/CLOCK:−45 bp Per2 protein/DNA complex when compared with wild-type samples ( Fig. 2k,l ). Adding recombinant p53 to the p53 −/− nuclear extract reduced the level of the BMAL1/CLOCK:−45 bp Per2 DNA complex ( Fig. 2m ). This observation shows that p53 competes with BMAL1/CLOCK for binding to the DNA probe. Collectively, these studies show that the Per2 promoter contains a functional p53 response element that overlaps with the E-box for BMAL1/CLOCK binding, which is critical for transcription of the Per2 gene. p53 levels regulate Per2 transcription in the SCN To gain insight into the relevance of the p53 response element in the Per2 promoter to clock function, p53 levels in the SCN, the master clock structure in mammals, were investigated under temporal conditions. Previous studies have shown that in peripheral tissues, the p53 protein level is under temporal control [23] , [24] , [25] . Immunofluorescence analysis with anti-p53 antibodies showed that the level of p53 in the SCN from wild-type mice peaks at ZT4–ZT8 and reaches a nadir at ZT16–ZT20 ( Fig. 3a,b ). There was no p53 staining in the SCN of p53 −/− mice. This observation is consistent with results from the ChIP assay that showed peak levels of p53 binding to the Per2 promoter occurred at about ZT4–ZT8. 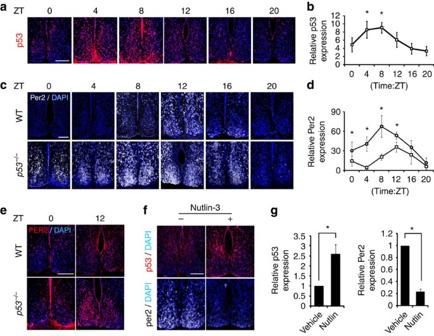Figure 3: p53 oscillates and modulatesPer2expression in the SCN. (a) Immunofluorescence analysis of p53 expression in WT mouse SCN. (b) Quantification of p53 expression in the SCN (n=3). ANOVA:P<0.05.post hoc t-test: *P<0.05. (c)In situhybridization detection ofPer2mRNA in SCN of WT andp53−/−mice. (d) Quantification ofPer2expression in the WT (square) andp53−/−(circle) mouse SCN (n=3). ANOVA:P<0.05.post hoc t-test: *P<0.05. (e) Immunofluorescence analysis of PER2 expression in SCNs from WT orp53−/−mice (f) Correlation between p53 protein levels, shown by immunofluorescence, andPer2expression, shown byin situhybridization, in Nutlin-3 (200 mg kg−1) or DMSO-injected SCN. (g) Statistical analysis off(n=2). Scale bars, 200 μm. Error bars: mean±s.e.m.t-Test: *P<0.05. Figure 3: p53 oscillates and modulates Per2 expression in the SCN. ( a ) Immunofluorescence analysis of p53 expression in WT mouse SCN. ( b ) Quantification of p53 expression in the SCN ( n =3). ANOVA: P <0.05. post hoc t -test: * P <0.05. ( c ) In situ hybridization detection of Per2 mRNA in SCN of WT and p53 −/− mice. ( d ) Quantification of Per2 expression in the WT (square) and p53 −/− (circle) mouse SCN ( n =3). ANOVA: P <0.05. post hoc t -test: * P <0.05. ( e ) Immunofluorescence analysis of PER2 expression in SCNs from WT or p53 −/− mice ( f ) Correlation between p53 protein levels, shown by immunofluorescence, and Per2 expression, shown by in situ hybridization, in Nutlin-3 (200 mg kg −1 ) or DMSO-injected SCN. ( g ) Statistical analysis of f ( n =2). Scale bars, 200 μm. Error bars: mean±s.e.m. t -Test: * P <0.05. Full size image Next, we examined whether the loss of p53 elevates Per2 expression in the SCN as predicted by our in vitro studies. In situ hybridization studies showed that Per2 transcript levels in the SCN of p53 −/− mice were significantly elevated compared with wild-type mice at most sampling times ( Fig. 3c,d ). Interestingly, the expression of Per2 transcripts in p53 −/− mice remained under temporal control and was apparently phase advanced, reaching peak levels at about ZT8 and a nadir at about ZT20. Consistent with results from in situ analysis, immunofluorescence studies with anti-PER2 antibodies showed that the level of PER2 was significantly elevated at ZT0 and ZT12 in the SCN of p53 −/− mice compared with wild-type mice ( Fig. 3e ). Next, we examined whether increasing p53 protein levels by Nutlin-3 treatment would have the converse effect of repressing Per2 transcription in the SCN. First, we investigated whether Nutlin-3 could stabilize p53 levels in the SCN. Wild-type mice were administered Nutlin-3 or vehicle (dimethylsulphoxide (DMSO)) at ZT9 and then killed at ZT14. We selected ZT14 for these studies as endogenous SCN Per2 and p53 protein levels are close to their peak and nadir, respectively, at this time point. Immunofluorescence analysis with anti-p53 antibodies showed increased p53 protein in the SCN after treatment with Nutlin-3 but not vehicle ( Fig. 3f,g ). In situ hybridization with an antisense Per2 probe showed that endogenous Per2 expression in the SCN of mice treated at ZT14 was significantly dampened after treatment with Nutlin-3 compared with vehicle ( Fig. 3f,g ). Thus, in the SCN, increased p53 levels lead to repression of Per2 expression, consistent with the finding of elevated Per2 expression in p53 −/− mice. p53 modulates the circadian behaviour of mice Next, we examined whether p53 regulates the circadian rhythm behaviour of mice. The circadian behaviour of inbred male p53 −/− and wild-type (C57BL/6) mice was analysed by monitoring their wheel-running activity. Both p53 −/− and wild-type mice entrained to an light-dark (LD) cycle and were rhythmic throughout our studies. The p53 −/− mouse period lengths were 22.8±0.1 h (mean±s.e.m., n =12) and were significantly shorter than wild-type period lengths of 23.3±0.1 h (mean±s.e.m., n =10) ( Fig. 4a,b ). In addition, the p53 −/− mice had a more widely distributed period that exhibited sudden and unpredictable changes during free-running conditions ( Fig. 4a,c ). To assess this phenotype further, the same p53 −/− and wild-type mice were re-entrained to an LD cycle followed by a second release into free-running conditions. For wild-type mice, the changes in period measured from the second release into dark-dark (DD) cycle were all within 0.06±0.01 h (mean±s.e.m., n =8) of their first measurements. In contrast, p53 −/− mice had periods that differed significantly from the first measurement ( Fig. 4c,d ). Both lengthening and shortening of periods were observed. Comparing the longest and shortest period length of an individual mouse measured by linear regression sampled over at least 10 days revealed an average difference of 0.43±0.1 h (mean±s.e.m., n =7) for p53 −/− mice. 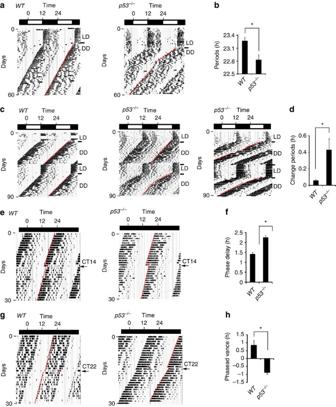Figure 4: p53 controls circadian behaviour of mice. (a,c) Wheel-running activity of WT andp53−/−mice. (b) Summary of periods for WT (n=10) andp53−/−mice (n=13). (d) Average difference in observed period length after re-entrainment of individual WT (n=8) andp53−/−(n=7) mice. (e) A 15-min light pulse applied at CT14 to the free-running mice. (f) Summary ofe: WT (n=3) andp53−/−(n=4). (g) A 15-min light pulse applied at CT22 to free-running mice. (h) Summary ofg: WT (n=3) andp53−/−(n=5). Error bars, mean±s.e.m.t-Test: *P<0.05. Figure 4: p53 controls circadian behaviour of mice. ( a , c ) Wheel-running activity of WT and p53 −/− mice. ( b ) Summary of periods for WT ( n =10) and p53 −/− mice ( n =13). ( d ) Average difference in observed period length after re-entrainment of individual WT ( n =8) and p53 −/− ( n =7) mice. ( e ) A 15-min light pulse applied at CT14 to the free-running mice. ( f ) Summary of e : WT ( n =3) and p53 −/− ( n =4). ( g ) A 15-min light pulse applied at CT22 to free-running mice. ( h ) Summary of g : WT ( n =3) and p53 −/− ( n =5). Error bars, mean±s.e.m. t -Test: * P <0.05. Full size image Phase shift behaviour in response to a light pulse of a specific circadian time (CT) is an intrinsic clock control behaviour [26] . Mice in the free-running state were given a 15-min light pulse at either CT14 or CT22 to measure their phase delay or phase advance response, respectively. The level of phase delay in response to a CT14 light pulse averaged −1.4±0.1 h (mean±s.e.m., n =3) in wild type, whereas p53 −/− mice displayed a significantly enhanced phase delay response that averaged −2.3±0.1 h (mean±s.e.m., n =4) ( Fig. 4e,f ). When the light pulse was given at CT22, wild-type mice displayed a phase advance response that averaged +0.8 h±0.3 h (mean±s.e.m., n =3). Surprisingly, the p53 −/− mice displayed no phase advance but instead exhibited a phase delay response that averaged −0.9 h±0.1 h (mean±s.e.m., n =5) ( Fig. 4g,h ). Thus, the circadian period of p53 −/− compared with wild-type mice is shorter, unstable and its phase shift response to a light cue displays an enhanced phase delay response during free-running conditions. Nutlin-3 phase shifts the circadian behaviour of mice Nutlin-3 is currently in clinical trials as an anti-cancer drug [27] . Preclinical studies showed that Nutlin-3 has apparent low toxicity and can be given daily to mice [17] . Our molecular studies raised the possibility that Nutlin-3 can alter Per2 expression via stabilization of p53 and thus reset the circadian clock. To investigate this possibility, we examined whether Nutlin-3 or vehicle (DMSO) can phase shift circadian rhythm in wild-type mice during free-running DD conditions. CT9 and CT21 were chosen due to the approximate peak and nadir levels of endogenous p53 in the SCN, respectively. Both vehicle- and Nutlin-3-treated mice displayed a temporary reduction of locomotor activity, although the effect of Nutlin-3 persisted longer in some animals. However, no phase shift response was observed in vehicle-treated wild-type or Nutlin-3-treated p53 −/− mice, whether treated at CT9 or CT21 ( Fig. 5a,b and Supplementary Fig. S6 ). In contrast, a phase advance response was observed when wild-type mice were treated with Nutlin-3 at CT9 or CT21. The effect of Nutlin-3 was also examined using a different protocol for phase shift response in the presence of a lighting cue. In this protocol, the delivery of vehicle or Nutlin-3 was carried out on the last day of the LD cycle entrainment followed by free-running conditions [28] . This protocol showed that vehicle-treated mice did not display phase shift behavior, whereas Nutlin-3 given at ZT9 induced a robust phase advance response ( Fig. 5c–e ). In contrast, p53 −/− mice treated with vehicle or Nutlin-3 displayed no phase shift response. These results show that the clock phase advance induced by Nutlin-3 treatment is mediated through stabilization of p53 and is consistent with light pulse studies of p53 −/− mice showing enhanced phase delay response. 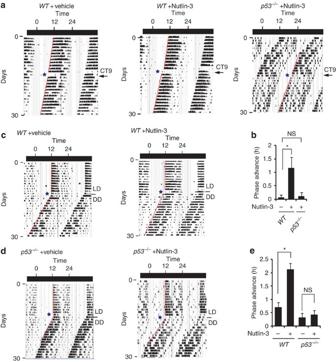Figure 5: Actograms of phase shift response induced by Nutlin-3. (a) WT orp53−/−mice were kept in a DD cycle and either vehicle (DMSO) (n=3) or Nutlin-3 (n=6) was injected at CT9. (b) Summary of phase advance (CT9). (c) Mice were kept in a 12 h/12 h LD cycle for 2 weeks, vehicle (n=6) or Nutlin-3 (n=4) were injected and then mice were released into a DD cycle. (d)p53−/−mice given vehicle (n=5) or Nutlin-3 (n=6), as inc. (e) Summary of phase advance of vehicle (−) or Nutlin-3 (+)-injected mice. Error bars, mean±s.e.m.t-test: *P<0.05. NS, not significant. Figure 5: Actograms of phase shift response induced by Nutlin-3. ( a ) WT or p53 −/− mice were kept in a DD cycle and either vehicle (DMSO) ( n =3) or Nutlin-3 ( n =6) was injected at CT9. ( b ) Summary of phase advance (CT9). ( c ) Mice were kept in a 12 h/12 h LD cycle for 2 weeks, vehicle ( n =6) or Nutlin-3 ( n =4) were injected and then mice were released into a DD cycle. ( d ) p53 −/− mice given vehicle ( n =5) or Nutlin-3 ( n =6), as in c . ( e ) Summary of phase advance of vehicle (−) or Nutlin-3 (+)-injected mice. Error bars, mean±s.e.m. t -test: * P <0.05. NS, not significant. Full size image The circadian clock mechanism governs the rhythmic activities that allow a living organism to anticipate and respond to opportunities and challenges presented in a daily manner. For this coordinated control to happen at all levels, from physiological processes to molecular signalling pathways, there must be a pervasive and effective mechanistic connection between the clock network and other cellular networks. It is now recognized that the clock mechanism or specific components of the clock are involved in responses to cellular stress including DNA damage response, checkpoint arrest and apoptosis [29] . p53-regulated genes are involved in diverse biological pathways including the cell cycle, DNA damage response, apoptosis and glucose metabolism [4] . However, the link between p53-controlled pathways such as the cell cycle and the circadian clock regulators is thought to be indirect or ‘opportunistic’ [30] . Our present study has shown that p53 directly binds to the Per2 promoter and represses its transcriptional activation by BMAL1/CLOCK. We mapped a p53 response element with two characteristic decamers to an evolutionarily conserved region within the −45 bp of the Per2 promoter transcription start site. This p53 response element overlaps with the major E-box element necessary for BMAL1/CLOCK-mediated transcription. Both EMSA and reporter assay with −45 bp Per 2DNA demonstrate p53 binding and repression of BMAL1/CLOCK-mediated transcription. Independently, by ChIP–qPCR analysis, we showed that BMAL1/CLOCK binding to the Per2 promoter is inhibited by the expression of p53. Four modes of p53 transcriptional repression are now recognized [20] . One of these modes is the overlap of the p53 response element with the binding site of another transcription factor, allowing p53 to compete with that transcription factor for DNA binding ( Fig. 6 ). Consistent with this mode of transcriptional repression, EMSA results show that the formation of a BMAL1/CLOCK:−45 bp Per2 DNA complex was significantly reduced by the addition of recombinant p53. 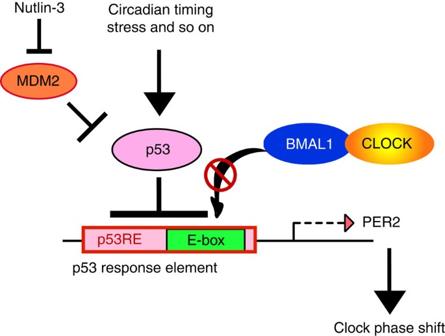Figure 6: Model of p53 repression ofPer2expression and modulation of the circadian clock. p53 levels are regulated by many factors such as circadian timing, cellular stress and MDM2. Both physiological and stress-induced p53 binds to the p53 response element of thePer2promoter, which overlaps with the BMAL1/CLOCK-binding site (E-box) and suppresses BMAL1/CLOCK-mediated transcription ofPer2, thereby modulating the circadian clock. Figure 6: Model of p53 repression of Per2 expression and modulation of the circadian clock. p53 levels are regulated by many factors such as circadian timing, cellular stress and MDM2. Both physiological and stress-induced p53 binds to the p53 response element of the Per2 promoter, which overlaps with the BMAL1/CLOCK-binding site (E-box) and suppresses BMAL1/CLOCK-mediated transcription of Per2 , thereby modulating the circadian clock. Full size image Our studies show that the physiological p53 level oscillates in the SCN of wild-type mice with peak expression around ZT8. In the SCN of p53 −/− mice, Per2 expression was significantly elevated but remained under temporal control. These observations suggest that p53 regulates the amplitude of Per2 transcription. Indeed, the p53 response element of the Per2 promoter is within a region previously delineated to be important for the generation of amplitude [21] . The p53 −/− mice display abnormal circadian behaviour, exhibiting a shorter period length with reduced precision and altered phase shift response to a light pulse. Interestingly, transgenic mice that overexpress Per2 also display a shorter period length than wild-type mice [31] . Period length is also controlled by PER2 phosphorylation state as it regulates the PER2 turnover [32] . Our current findings show that when the levels of p53 are elevated by Nutlin-3 treatment, by γ-irradiation or by expression construct transfection in cultured cells, Per2 expression is significantly dampened. In the in vivo study, Nutlin-3 injection into mice produced elevated p53 protein and repressed Per2 expression in the SCN, resulting in phase advancement of the circadian clock. These findings suggest that both physiological and elevated levels of p53 regulate Per2 expression. The importance of physiological levels of p53 for other biological processes has been recently recognized. For example, physiological levels of p53 regulate CD44 expression and epithelial proliferation [33] . In addition, under non-stress conditions, p53 regulates adult neural stem cell proliferation [34] . Under stress conditions, stabilized p53 represses the expression of Per2 , which in turn could modulate the expression of other clock genes to help reset the clock. BMAL1/CLOCK-mediated Per1 and Cry1 expressions also seem to be repressed by p53 ( Supplementary Fig. S7 ), though it is unclear whether these genes are direct targets of p53 inhibition or whether this is secondary to Per2 repression by p53. It was previously shown that loss of PER2 leads to highly dampened Per1 and Cry1 expression in vivo [35] . This study shows that p53 −/− mice displayed an increased phase delay and an absence of phase advance response to a light pulse at CT14 and CT22, respectively. Mice deficient in PER2 function exhibited enhanced phase advance and a weak phase delay response, indicating that PER2 has a major role in phase shift control [36] , [37] , [38] . Per2 expression is differentially induced by light over the span of the phase response curve. A light pulse given during early, but not late subjective night, induced Per2 expression in the SCN [36] , [37] . These observations suggest that relative to the phase response curve, increased induction of PER2 is associated with phase delay, whereas a lack of induction of PER2 is associated with the phase advance response. This correlation of rapid reduction of PER2 levels with phase shift advance is supported by cell culture studies showing that DNA damage induced by methyl methane sulphonate (MMS) or ultraviolet irradiation caused clock phase advancement as a result of a rapid decrease in PER2 levels [39] . Genotoxic agents such as ultraviolet or γ-irradiation rapidly induce p53 (refs 19 , 24 , 40 ). Our studies show that γ-irradiation caused rapid p53 stabilization, which was associated with decreased PER2 levels. This decline in PER2 was not observed in p53 −/− MEF treated with γ-irradiation, indicating that it is a p53-dependent effect. Consistent with these findings, mice treated with γ-irradiation also displayed phase advancement of their circadian clock [41] . Conversely, it has been observed that casein kinase 1 inhibitors when given during free-running conditions induce a phase delay response in mice [42] . This phase shift effect of casein kinase 1 inhibitors is thought to be caused by increased stabilization of PERIOD proteins, particularly PER2 (refs 42 , 43 ). Our observation that Nutlin-3 induced p53-mediated repression of Per2 expression and phase advancement of the clock is consistent with a phase advance response resulting from a reduced induction of PER2 levels by a light pulse at ZT22. Previously, it had been observed that mice heterozygous for constitutively active p53 displayed an enhanced aging phenotype that included enhanced loss of soft tissues and development of spinal kyphosis [44] . Further, overactive p53 activities caused by the expression of the p53 isoform ΔN-p53 (p44) also resulted in a similar premature ageing phenotype [45] , [46] . Interestingly, similar premature ageing phenotypes, including progressive loss of soft tissues and spinal kyphosis, were observed in Per2 -deficient mice [47] , [48] . These premature ageing phenotypes in hyperactive p53 and Per2 −/− mice are supportive of our findings that p53 suppresses Per2 expression. Current evidence suggests that there is an inter-regulatory loop between p53, PML and Per 2. PML is involved in the regulation p53 acetylation and function [14] , [15] . However, PML is a p53 target [49] . Both p53 and PML are under circadian control [6] , [25] . Our studies showed PML and p53 can directly regulate the circadian clock via Per 2. Clearly, the mechanistic detail of their inter-regulation is complex and remains to be fully deciphered. In summary, our earlier study suggested that functional PER2 is important for p53-mediated stress signals to reach the circadian clock network [24] . Here we show that p53 acts as a transcription factor that regulates the circadian clock by direct control of Per2 expression. Animals p53 −/− (C57BL/6) mice were obtained from The Jackson Laboratory (cat. no. 002101). Animals were housed in a standard animal maintenance facility under a 12-h light: 12-h dark cycle. All animal studies were carried under institutional approved animal protocols (HSC-AWC-09-139). Cells and reagents WT MEF cells and Trp53 −/− MEF cells were obtained from Dr. C. Takahashi (Kanazawa University, Japan) and maintained in DMEM/10% FCS. Nutlin-3 was purchased from Cayman Chemical (cat. no. 10009816). The mouse p53 expression vector was purchased from ORIGENE. A mouse anti-α-tubulin monoclonal antibody was purchased from COVANCE (B-5-1-2). The mPer2 antibody was raised as described previously [35] . Anti-p53 antibodies are from Santa Cruz (FL-393, cat. no. sc-6243, DO-1, cat. no. sc-126) and from Calbiochem (PAb421, cat. no. OP03). The anti-BMAL1 antibody is from Abcam (ab3350). The anti-CLOCK antibody is from Thermo Scientific (PA1-520). The anti-Lamin A antibody is from BD Transduction Laboratories (cat. no.612162). mPer2- promoter Luc reporter constructs including −2,811, −1,982, −661, −386, −105 were kind gifts from Dr. T. Takumi [21] . The −105 bp Per2 -luc reporter construct containing five point mutations was generated by two-step site-directed mutagenesis using QuikChange Site-Directed Mutagenesis Kit (cat. no. 200519, Stratagene). An intermediate mutant was created by introducing two mutations to the p53-binding motif in the Per2 promoter using an oligonucleotide with the sequence 5′-GCGCGCGCAGGGGAGGACTCAGCGCGCGC-3′. Then, an additional three mutations were introduced to the same motif using an oligonucleotide with a sequence of 5′-CCAATGGCGCGCGCAGTTGAGGACACAGCGCGCGCGG-3′. Luciferase reporter assay Luciferase reporter assays were performed as previously described [50] . Briefly, MEF cells were seeded into 12-well plates and transfected with the Per2 luciferase reporter construct or the Bmal1 luciferase reporter construct using the Lipofectamine 2000 (Invitrogen). Co-transfections were performed with the respective expression constructs for Clock , Bmal1, Rorα and p53 Cells were harvested 24 h post transfection, and luciferase assay was performed with an assay kit obtained from Promega using a TD-20/201 luminometer (Turner Designs). Immunoblotting Cells were lysed in ice-cold lysis buffer containing 50 mM Tris-HCl, pH 7.4, 0.1% SDS, 0.25 mM deoxycholate, 150 mM NaCl, 2 mM EGTA, 0.1 mM Na 3 VO 4 , 10 mM NaF, 1 mM PMSF and complete protease inhibitor (Roche). The cell lysates were resolved by SDS–PAGE and used for immunoblotting, as described previously [51] . Briefly, the first antibody incubation for immunoblotting was performed at 4 °C overnight in the blocking buffer (5% milk, 1% goat serum, Tris-Buffered Saline with 0.1% Tween 20 (TBS-T)). The antibodies dilution we used were anti-mPer2 (150,000 × ), anti-p53 (10,000 × ), anti-alpha-tubulin (10,000 × ) and anti-Lamin A (2,500 × ). Electric mobility shift assay EMSA was carried out using a Light-Shift Chemiluminescent EMSA kit (cat. no. 20148, PIERCE) as described previously [52] . Briefly, the following double-stranded 5′-biotinylated or unlabelled DNAs were synthesized (SIGMA Aldrich); Per2 consensus sequence DNA: 5′-CAGGGGCGGGCTCAGCGCGCGCGGTCACGTTTTCCACTATGTGACAGCGGAGG-3′, Per2 mutant promoter DNA: 5′-CAGTTGAGGACACAGCGCGCGCGGTCACGTTTTCCACTATGTGACAGCGGAGG-3′. Per2 consensus −55 bp oligo: 5′-ATGGCGCGCGCAGGGGCGGGCTCAGCGCGCGCGGTCACGTTTTCCACTATGTGACAGCGGAGG-3′, Per2 mutant consensus −55 bp oligo: 5′- ATGGCGCGCGCAGTTGAGGACACAGCGCGCGCGGTCACGTTTTCCACTATGTGACAGCGGAGG-3′. Recombinant mouse p53 was purchased from Active Motif (cat. no. 31103) and 2 ng of recombinant p53 was used per reaction. Binding assays were performed in a buffer containing 20 mM HEPES (pH 7.6), 30 mM KCl, 1 mM EDTA, 10 mM (NH 4 ) 2 SO 4 , 1 mM DTT, 0.2% Tween-20, 1 μg poly [d(A-T)], 0.1 μg poly L -lysine. Anti-p53 antibodies (pAb421, Calbiochem or DO-1, Santa Cruz) were used for super-shift assay. For BMAL1/CLOCK binding assay, nuclear extracts were prepared as described previously [53] . Briefly, cells were washed once with Buffer A containing 10 mM HEPES (pH 7.3), 1.5 mM MgCl 2 , 10 mM KCl and 0.5 mM DTT, and resuspended in Buffer A. Cells were homogenized, centrifuged (200 r.p.m., 10 min) and nuclei were washed again with Buffer A. Cell pellets were resuspended in Buffer C containing 20 mM HEPES (pH 7.3), 20% glycerol, 0.42 M NaCl, 1.5 mM MgCl 2 , 0.2 mM EDTA, 0.5 mM DTT, 0.5 mM phenylmethylsulfonyl fluoride and protease inhibitor cocktail (Roche). Lysates were incubated for 30 min with constant rotation at 4 °C and centrifuged (8,000 r.p.m., 10 min). Supernatants were used as nuclear extracts. Binding assays were performed in a buffer containing 50 mM Tris-HCl (pH 8.0), 100 mM KCl, 1 mM EDTA, 6 mM DTT and 1 μg poly [d(A-T)] [54] . The anti-BMAL1 antibody (N-20, 2 μg, Santa Cruz) and anti-FLAG M2 antibody (5 μg, SIGMA) were used to detect the specific BMAL1/CLOCK band. The anti-BMAL1 antibody was previously validated by other investigators [55] . Protein binding reactions were performed in 10 μl scale. Chromatin immunoprecipitation assay ChIP assay was performed as described previously [56] . Briefly, cells or tissues were fixed with 1% formalin for 10 min. Crosslinking was stopped by adding 125 mM glycine. Cells were washed and homogenized using a homogenizer. Homogenized cells were collected by brief centrifugation and lysed with swelling buffer containing 5 mM PIPES (pH 8.0), 85 mM KCl, 1% NP40 and protease inhibitor cocktail (cat. no. 11697498001, Roche). Nuclear fractions were collected by centrifugation and lysed with nuclear lysis buffer containing 50 mM Tris-HCl (pH 8.0), 10 mM EDTA, 1% SDS and protease inhibitor cocktail. Sonication was performed to fragment DNA to ~500 bp. After centrifugation, lysates were precleared with protein A agarose (Invitrogen). Precleared samples were diluted with the same volume of immunoprecipitation (IP) dilution buffer containing 16.7 mM Tris-HCl (pH 8.0), 0.01% SDS, 1.1% Triton X-100, 1.2 mM EDTA, 167 mM NaCl and protease inhibitor cocktail. Then, p53 and BMAL1 were immunoprecipitated with anti-p53 antibody (2 μg, sc-6243) or anti-BMAL1 antibody (2 μg, ab3350, abcam) and collected on protein A agarose. After serial washing with dialysis buffer containing 50 mM Tris-HCl (pH 8.0), 2 mM EDTA and 0.2% sarkosyl, and IP wash buffer containing 100 mM Tris-HCl (pH9.0), 500 mM LiCl, 1% NP40, 1% Deoxycholate and protease inhibitor cocktail; p53–DNA complexes were eluted by elution buffer containing 50 mM NaHCO 3 and 1% SDS. Eluted samples were mixed with 0.2 M NaCl and incubated at 67 °C overnight, then RNase A treated and purified. PCR and quantitative real-time PCR were performed using Per2 -Ebox2 forward primers: 5′-CAGGTTCCGCCCCGCCAGTAT-3′, reverse primer:5′-GTCGCCCTCCGCTGTCACATAG-3′ and Per2 -Ebox5 forward primer: 5′-CTCTGTAGGGTGGAGCGGCGA-3′, reverse primer: 5′-ATCCCCACTGCTCCTTCGCAC-3′. ChIP samples obtained from SCN and thymus were analysed by real-time PCR (ABI PRISM 7700 system, Applied Biosystems) using Maxima SYBR Green qPCR Master Mix (cat. no. 0252, Fermentas). Real-time PCR data were analysed as previously reported [57] . IgG control antibody was used as a negative control. Δ C t was obtained by C t experiment sample − C t negative control and fold differences were calculated by [2 (−Δ C t) ]. Immunofluorescence staining Mouse brains from 8–10-week-old WT and Tr p53 −/− were collected at the indicated time point, fixed with 4% PFA and embedded in paraffin. Then 8 μm sections were obtained and stained with anti-p53 antibody (cat. no. sc-6243, 50 × , SantaCruz), or anti-mPER2 antibody (4,000 × ) and visualized by secondary anti-rabbit IgG Alexa Fluor 555 antibody (cat. no. A21429, 1,000 × , Invitrogen). In situ hybridization 8–10 week old WT and Tr p53 −/− mouse brains were collected at the indicated time point, fixed with 4% PFA, and embedded in paraffin. Then 8 μm sections were obtained and in situ hybridization was performed as described previously [58] with some modifications. Briefly, paraffin sections were treated with 1 μg ml −1 protease K in PBS-T (0.1% Tween-20) at 37 °C for 15 min, washed, fixed with 4% performic acid at room temperature for 15 min, washed, and then incubated with digoxigenin-labeled cRNA probes in buffer containing 50% formamide, 1% SDS, 5 × SSC, 50 μg ml −1 tRNA, and 20 μg ml −1 heparin at 55 °C overnight. The probe for Per2 was described previously [59] . Hybridized sections were washed with Buffer A containing 50% formamide, 1% SDS, and 5 × SSC twice at 55 °C for 30 min each and then washed with Buffer B containing 50% formamide and 2 × SSC three times at 55 °C for 30 min each. After washing with TBS-T (pH 7.6, 0.1% Tween-20) three times, sections were blocked with 0.5% blocking reagent (cat. no. 11096176001, Roche) for 1 h and incubated with anti-alkaline phosphatase-conjugated anti-DIG antibody (cat. no. 11093274910, 1000 × , Roche) at 4 °C overnight. Sections were washed three times with TBS-T and immersed in NTMT (NaCl Tris MgCl 2 Tween 20) buffer containing 100 mM Tris-HCl (pH 9.5), 100 mM NaCl, 50 mM MgCl 2 , 0.1% Tween-20, and 2 mM levamisol. Sections were then developed with NBT/BCIP reagents. Locomoter activity Wheel-running activity was monitored as described [60] . Male wild type and Trp53 −/− mice aged about 4 weeks were used. Nutlin-3 (200 mg kg −1 ) or vehicle (DMSO) was injected intraperitoneally at the indicated time point. How to cite this article: Miki, T. et al. p53 regulates Period2 expression and the circadian clock. Nat. Commun. 4:2444 doi: 10.1038/ncomms3444 (2013).